p47 negatively regulates IKK activation by inducing the lysosomal degradation of polyubiquitinated NEMO The persistent or excess activation of NF-κB causes various inflammatory and autoimmune diseases, but the molecular mechanisms that negatively regulate NF-κB activation are not fully understood. Here we show that p47, an essential factor for Golgi membrane fusion, associates with the NEMO subunit of the IκB kinase (IKK) complex upon TNF-α or IL-1 stimulation, and inhibits IKK activation. p47 binds to Lys63-linked and linear polyubiquitin chains, which are conjugated to NEMO upon such stimulation. The binding of p47 to polyubiquitinated NEMO triggers the lysosomal degradation of NEMO, thereby inhibiting IKK activation. The silencing of p47 results in enhanced TNF-α- or IL-1-induced IKK activation, and an increased expression of genes encoding inflammatory mediators. Taken together, our results suggest that p47 is critical for negatively regulating stimulation-induced IKK activation in a manner that is mechanistically distinct from the previously characterized negative regulators, such as A20 and CYLD. The post-translational modification of proteins is crucial for the regulation of various intracellular signal transduction pathways. Recent studies have clearly demonstrated that in addition to phosphorylation, ubiquitination is a strategy for regulating biologically important pathways such as those that activate transcription factor nuclear factor-κB (NF-κB) [1] , [2] , [3] . NF-κB is a dimeric transcription factor formed by the Rel/NF-κB family members, including p50, p52, RelA, RelB and c-Rel, and it has crucial roles in immune responses, inflammation, cell proliferation and survival [4] . NF-κB is sequestered in the cytoplasm via its association with inhibitory proteins of the κB family (IκBs) or NF-κB precursors, such as p100 and p105, the C termini of which contain IκB-like ankyrin repeats. The classical NF-κB pathways are activated by cytokines, such as tumour necrosis factor (TNF)-α and interleukin (IL)-1, and bacterial products. Stimulation with these ligands leads to the activation of the IκB kinase (IKK) complex, which consists of the catalytic subunits IKKα and IKKβ, and the regulatory subunit NF-κB essential modulator (NEMO). IKK then phosphorylates IκBs and targets them for Lys48-linked polyubiquitination, which leads to the degradation of ubiquitinated IκBs by the proteasome, allowing NF-κB to enter the nucleus and activate target genes [3] . Alternatively, the non-classical pathways, which are activated by stimulation from CD40, receptor activator of NF-κB or lymphotoxin-β receptor, involve the proteasome-dependent selective degradation of the C-terminal ankyrin repeats of p100 (ref. 5 ). In the IL–1R pathway, IKK activation requires the generation of unanchored Lys63-linked polyubiquitin chains [6] or their conjugation to TNF receptor-associated factor (TRAF)-6 (ref. 7 ) and transforming growth factor-β-activated kinase (TAK)-1 (ref. 8 ), both of which are catalysed by TRAF6 (E3) and the Ubc13/Uev1A complex (E2) [9] . These Lys63-linked polyubiquitin chains do not induce proteasomal degradation but act as platforms for the formation of active signal complexes that consist of MEKK3, TAK1, TAK1-binding (TAB) 2/TAB3 and the IKK complex, because TAB2/3 and NEMO bind to Lys63-linked polyubiquitin chains via their ubiquitin-binding domains [8] , [10] , [11] . This complex formation leads to the activation of TAK1, which then phosphorylates and activates IKKβ [9] , [12] . Upon TNF-α stimulation, TNF receptor-1 recruits the adaptor TRADD, the E3 ubiquitin ligases TRAF2 and cIAPs, and the kinase RIP1, which results in the polyubiquitination of RIP1 (refs [13] , [14] , [15] ). The polyubiquitin chain of RIP1 also acts as a platform for the formation of an active TAK1-containing complex. In addition to TAK1 activation, IKK activation requires the stimulation-induced conjugation of Lys63-linked or linear polyubiquitin chains to NEMO [2] , [16] , [17] , [18] , [19] , which may induce oligomer formation or a conformational change in NEMO to activate the IKK complex [1] . The former conjugation is catalysed by TRAF6 and the latter by the linear ubiquitin chain assembly complex, which is composed of HOIL-1, HOIP and Sharpin [20] , [21] , [22] . Given that the persistent or excess activation of NF-κB promotes chronic inflammation, autoimmunity and malignancy [23] , [24] , [25] , [26] , IKK activation needs to be tightly regulated, which highlights the physiological significance of IKK-negative regulators. Among these regulators, two deubiquitinases (DUBs), CYLD and A20, disassemble Lys63-linked or linear polyubiquitin chains, thereby negatively regulating IKK [27] , [28] , [29] , [30] . As these two proteins act through distinct molecular mechanisms, they function non-redundantly and their inactivation leads to serious disorders [25] , [31] . Thus, the polyubiquitin-chain-targeted negative regulation of IKK is crucial for homeostasis. In the present study, we identified p47 (also known as NSFL1C) [32] , a major adaptor of the cytosolic ATPase associated with various cellular activities p97 (ref. 33 ), as a negative regulator of NF-κB activation. The p47/p97 complex is required for the reassembly of Golgi stacks at the end of mitosis [32] , [33] , [34] , [35] . Interestingly, p47 binds to NEMO upon TNF-α or IL-1 stimulation, and induces the lysosome-dependent degradation of polyubiquitinated NEMO without p97, thereby inhibiting IKK activation. Thus, we propose that p47 is involved in a previously unidentified mechanism for the polyubiquitin-chain-mediated negative regulation of NF-κB. The identification of p47 as a NEMO-binding protein To identify novel IKK regulators, we searched for proteins that bind to or dissociate from the IKK complex in a manner that is dependent on the Tax protein of the human T-cell leukaemia virus-1. The IKK complex was immunoprecipitated using an anti-Flag antibody from the cytosolic fraction of Jurkat cells that stably expressed Flag-NEMO following the addition of recombinant Tax to activate IKK [36] , and the proteins were analysed by mass spectrometry. Among the proteins identified, we focused on p47, because it binds to ubiquitinated proteins via its N-terminal ubiquitin-associated (UBA) domain [37] , [38] , [39] and is involved in the degradation of ubiquitinated proteins [40] , [41] . Moreover, we found that p47 is exclusively localized in the cytoplasm in various cell lines ( Supplementary Fig. S1 ), although p47 was previously reported to primarily localize to the nucleus in interphase and this was required for its inactivation [42] . A co-immunoprecipitation assay in HEK293T cells that transiently expressed HA–IKKα, IKKβ, or NEMO together with Flag-p47 revealed that NEMO bound to p47, whereas IKKα and IKKβ did not ( Fig. 1a ). To confirm the interactions under physiological conditions, we co-immunoprecipitated the endogenous proteins in HeLa cells. NEMO-bound p47 appeared after 5 min of stimulation with TNF-α ( Fig. 1b ) or IL-1 ( Fig. 1c ). These results indicate that p47 binds to the IKK complex through NEMO in a stimulation-dependent manner. 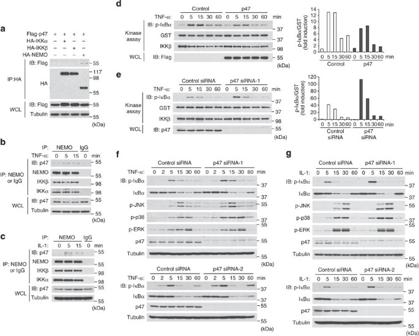Figure 1: The identification of p47 as a negative regulator of TNF-α- and IL-1-induced IKK activation. (a) HEK293T cells were transfected with a Flag-p47 expression plasmid (0.3 μg) together with a plasmid encoding HA-IKKα, HA-IKKβ or HA-NEMO (4 μg). Cell lysates were subjected to immunoprecipitation with an anti-HA antibody followed by immunoblotting with anti-HA and anti-Flag antibodies. Whole-cell lysate (WCL) was also prepared and analysed by immunoblotting with anti-Flag and anti-tubulin antibodies. (b,c) HeLa cells were treated with TNF-α (10 ng ml−1,b) or IL-1 (10 ng ml−1,c). Cell lysates were subjected to immunoprecipitation with a control IgG or anti-NEMO antibody followed by immunoblotting with the indicated antibodies. The WCL was analysed by immunoblotting with anti-p47 and anti-tubulin antibodies. (d) HEK293T cells were transfected with a control or a Flag-p47 expression plasmid. After 48 h, the cells were treated with TNF-α (10 ng ml−1). The IKK complex that had been immunoprecipitated with an anti-NEMO antibody was incubated at 30 °C for 1 h in a reaction mixture containing recombinant GST-IκBα (amino acids 1–54) followed by immunoblotting with anti-p-IκBα, anti-GST and anti-IKKβ antibodies. The relative activities of the IKK complex are expressed as the intensity of the band detected by the anti-p-IκBα antibody divided by the intensity detected by the anti-GST antibody. The intensities of the bands were quantified using ImageJ software (National Institutes of Health). (e) HEK293T cells were transfected with control or p47 siRNA-1. After 72 h, the cells were treated with TNF-α (10ng ml−1). The IKK kinase assay was performed as described ind. (f,g) HeLa cells were transfected with control, p47 siRNA-1 or p47 siRNA-2. After 72 h, the cells were treated with TNF-α (1 ng ml−1,f) or IL-1 (3 ng ml−1,g). The WCL was analysed by immunoblotting with the indicated antibodies. The depicted results are representative of three independent experiments. Figure 1: The identification of p47 as a negative regulator of TNF-α- and IL-1-induced IKK activation. ( a ) HEK293T cells were transfected with a Flag-p47 expression plasmid (0.3 μg) together with a plasmid encoding HA-IKKα, HA-IKKβ or HA-NEMO (4 μg). Cell lysates were subjected to immunoprecipitation with an anti-HA antibody followed by immunoblotting with anti-HA and anti-Flag antibodies. Whole-cell lysate (WCL) was also prepared and analysed by immunoblotting with anti-Flag and anti-tubulin antibodies. ( b , c ) HeLa cells were treated with TNF-α (10 ng ml −1 , b ) or IL-1 (10 ng ml −1 , c ). Cell lysates were subjected to immunoprecipitation with a control IgG or anti-NEMO antibody followed by immunoblotting with the indicated antibodies. The WCL was analysed by immunoblotting with anti-p47 and anti-tubulin antibodies. ( d ) HEK293T cells were transfected with a control or a Flag-p47 expression plasmid. After 48 h, the cells were treated with TNF-α (10 ng ml −1 ). The IKK complex that had been immunoprecipitated with an anti-NEMO antibody was incubated at 30 °C for 1 h in a reaction mixture containing recombinant GST-IκBα (amino acids 1–54) followed by immunoblotting with anti-p-IκBα, anti-GST and anti-IKKβ antibodies. The relative activities of the IKK complex are expressed as the intensity of the band detected by the anti-p-IκBα antibody divided by the intensity detected by the anti-GST antibody. The intensities of the bands were quantified using ImageJ software (National Institutes of Health). ( e ) HEK293T cells were transfected with control or p47 siRNA-1. After 72 h, the cells were treated with TNF-α (10ng ml −1 ). The IKK kinase assay was performed as described in d . ( f , g ) HeLa cells were transfected with control, p47 siRNA-1 or p47 siRNA-2. After 72 h, the cells were treated with TNF-α (1 ng ml −1 , f ) or IL-1 (3 ng ml −1 , g ). The WCL was analysed by immunoblotting with the indicated antibodies. The depicted results are representative of three independent experiments. Full size image p47 inhibits TNF-α- or IL-1-induced IKK activation To understand whether p47 affects IKK activation, we first examined the effect of p47 overexpression using in vitro kinase assays. TNF-α-induced IKK activation was significantly reduced by p47 overexpression ( Fig. 1d ), whereas p47 knockdown resulted in enhanced TNF-α-induced IKK activation ( Fig. 1e ). Moreover, p47 knockdown increased the phosphorylation and degradation of IκBα ( Fig. 1f,g ). The enhanced phosphorylation of IκBα by p47 knockdown was observed 5 min after TNF-α or IL-1 stimulation, consistent with the kinetics of the stimulation-induced association of p47 with NEMO ( Fig. 1b,c ). Although p47 is reported to be involved in various fundamental processes associated with cell division [32] , [33] , [34] , [35] , p47 knockdown had no effect on proliferation, survival or endoplasmic reticulum (ER) stress ( Supplementary Fig. S2 ), which strongly suggests that the enhanced NF-κB activation following p47 knockdown is not due to non-specific effects. Taken together, these results indicate that p47 negatively regulates TNF-α- and IL-1-induced IKK activation. p47 also inhibits Tax-induced IKK activation ( Supplementary Fig. S3 ). In addition, p47 knockdown slightly enhanced the TNF-α- and IL-1-induced activation of JNK and p38, but not that of ERK ( Fig. 1f,g ), which is consistent with the previous finding that NEMO is necessary for full JNK and p38 activation [43] . The lack of a significant effect of p47 knockdown on the level of phosphorylated p38 in non-stimulated cells suggests that cell stress is barely induced by p47 knockdown ( Fig. 1f,g ). p47 negatively regulates NF-κB-driven transcription To understand whether p47 affects the NF-κB-mediated transcription, we first checked the nuclear DNA-binding activity of NF-κB with an electrophoretic mobility shift assay. Nuclear NF-κB was significantly enhanced in p47-knockdown cells upon TNF-α and IL-1 stimulation ( Fig. 2a ). To measure the transcriptional activity of NF-κB, HEK293T cells were transfected with the NF-κB reporter plasmid, and the subsequent TNF-α stimulation- or p65 overexpression-induced luciferase activity was measured. p47 inhibited TNF-α-induced NF-κB activation in a dose-dependent manner but had no effect on p65-mediated transcription ( Fig. 2b,c ), indicating that p47 targets the IKK complex but has no effect on events that are downstream of IKK activation, such as the nuclear translocation or phosphorylation-mediated activation of p65 (ref. 44 ). As p47 knockdown resulted in a significant enhancement in TNF-α-induced NF-κB activity ( Fig. 2d ), we investigated the physiological significance of the p47-mediated negative regulation of NF-κB by measuring the expression levels of the NF-κB target genes. The TNF-α- or IL-1-induced expression of Il8 and Tnfa was notably enhanced in p47-knockdown cells ( Fig. 2e ), indicating that the p47-mediated negative regulation of IKK activation significantly affects NF-κB-driven transcription. 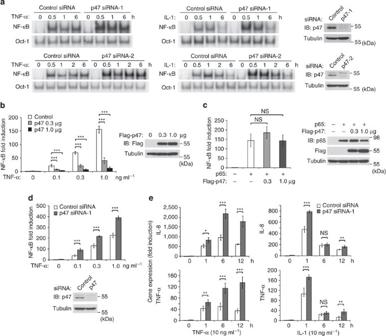Figure 2: p47 negatively regulates NF-κB-driven transcription. (a) HeLa cells that had been transfected with control, p47 siRNA-1 or p47 siRNA-2 were treated with TNF-α (10 ng ml−1) or IL-1 (10 ng ml−1). Nuclear extracts were subjected to electrophoretic mobility shift assay. The efficiency of p47 knockdown is shown. The depicted results are representative of three independent experiments. (b) HEK293T cells were transfected with a 3×κB-luc reporter and a Flag-p47 expression plasmid. The cells were treated with TNF-α for 24 h, and the resultant luciferase activity was measured. The fold induction was calculated by dividing each luciferase activity by that of the control without TNF-α stimulation. (c) HEK293T cells were transfected with a 3×κB-luc reporter and a p65 expression plasmid in combination with increasing amounts of a Flag-p47 expression plasmid. After 48 h, the subsequent luciferase activity was measured. The fold induction was calculated by dividing each luciferase activity by that of the control without p65 expression. (d) HEK293T cells were transfected with control or p47 siRNA-1. The cells were then transfected with a 3×κB-luc reporter and treated with TNF-α for 24 h, and the subsequent luciferase activity was measured. Fold induction was calculated by dividing each luciferase activity by that of the control siRNA treatment without TNF-α stimulation. (e) HeLa cells were transfected with control or p47 siRNA-1. After 60 h, the cells were treated with TNF-α or IL-1. The expression levels of IL-8 and TNF-α were measured by real-time RT–PCR. The fold induction was calculated by dividing each expression value by that of a control siRNA treatment without TNF-α or IL-1 stimulation. The results shown inb,c,dandeindicate the mean±s.d. (n=3). NS, not significant. Statistical significance was assessed using a Student'st-test. ***P<0.01, **P<0.02 and *P<0.05. Figure 2: p47 negatively regulates NF-κB-driven transcription. ( a ) HeLa cells that had been transfected with control, p47 siRNA-1 or p47 siRNA-2 were treated with TNF-α (10 ng ml −1 ) or IL-1 (10 ng ml −1 ). Nuclear extracts were subjected to electrophoretic mobility shift assay. The efficiency of p47 knockdown is shown. The depicted results are representative of three independent experiments. ( b ) HEK293T cells were transfected with a 3×κB-luc reporter and a Flag-p47 expression plasmid. The cells were treated with TNF-α for 24 h, and the resultant luciferase activity was measured. The fold induction was calculated by dividing each luciferase activity by that of the control without TNF-α stimulation. ( c ) HEK293T cells were transfected with a 3×κB-luc reporter and a p65 expression plasmid in combination with increasing amounts of a Flag-p47 expression plasmid. After 48 h, the subsequent luciferase activity was measured. The fold induction was calculated by dividing each luciferase activity by that of the control without p65 expression. ( d ) HEK293T cells were transfected with control or p47 siRNA-1. The cells were then transfected with a 3×κB-luc reporter and treated with TNF-α for 24 h, and the subsequent luciferase activity was measured. Fold induction was calculated by dividing each luciferase activity by that of the control siRNA treatment without TNF-α stimulation. ( e ) HeLa cells were transfected with control or p47 siRNA-1. After 60 h, the cells were treated with TNF-α or IL-1. The expression levels of IL-8 and TNF-α were measured by real-time RT–PCR. The fold induction was calculated by dividing each expression value by that of a control siRNA treatment without TNF-α or IL-1 stimulation. The results shown in b , c , d and e indicate the mean±s.d. ( n =3). NS, not significant. Statistical significance was assessed using a Student's t -test. *** P <0.01, ** P <0.02 and * P <0.05. Full size image p47 regulates IKK in a CYLD- and A20-independent manner We then addressed whether CYLD or A20 is involved in p47-mediated inhibition of IKK activation. The expression levels of CYLD and A20 were not affected by p47 knockdown at all time points tested ( Fig. 3a,b ), and p47 knockdown enhanced the phosphorylation of IκBα in Cyld - or A20 -deficient mouse embryonic fibroblast (MEF) cells ( Fig. 3c–f ). These results indicate that p47 inhibits IKK activation in an A20- and CYLD-independent manner. 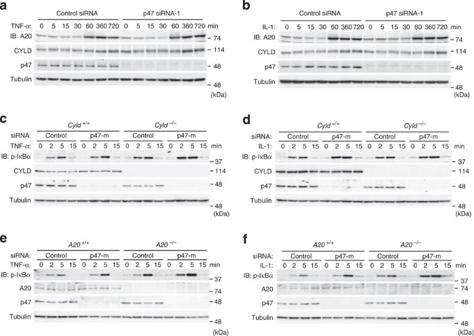Figure 3: p47 negatively regulates TNF-α- and IL-1-induced IKK activation independently of CYLD and A20. (a,b) HeLa cells were transfected with control or p47 siRNA-1. After 60 h, the cells were treated with TNF-α (10 ng ml−1,a) or IL-1 (10 ng ml−1,b) for the indicated times. The whole-cell lysate (WCL) was analysed by immunoblotting with the indicated antibodies. (c,d)Cyld+/+orCyld−/−MEFs were transfected with control or p47 siRNA-mouse. After 72 h, the cells were treated with TNF-α (3.0 ng ml−1,c) or IL-1 (3.0 ng ml−1,d) for the indicated times. The WCL was analysed by immunoblotting with the indicated antibodies. (e,f)A20+/+orA20−/−MEFs were transfected with control or p47 siRNA-mouse. After 72 h, the cells were treated with TNF-α (3.0 ng ml−1,e) or IL-1 (3.0 ng ml−1,f) for the indicated times. The WCL was analysed by immunoblotting with the indicated antibodies. p47-m, p47-mouse. The depicted results are representative of three independent experiments. Figure 3: p47 negatively regulates TNF-α- and IL-1-induced IKK activation independently of CYLD and A20. ( a , b ) HeLa cells were transfected with control or p47 siRNA-1. After 60 h, the cells were treated with TNF-α (10 ng ml −1 , a ) or IL-1 (10 ng ml −1 , b ) for the indicated times. The whole-cell lysate (WCL) was analysed by immunoblotting with the indicated antibodies. ( c , d ) Cyld +/+ or Cyld −/− MEFs were transfected with control or p47 siRNA-mouse. After 72 h, the cells were treated with TNF-α (3.0 ng ml −1 , c ) or IL-1 (3.0 ng ml −1 , d ) for the indicated times. The WCL was analysed by immunoblotting with the indicated antibodies. ( e , f ) A20 +/+ or A20 −/− MEFs were transfected with control or p47 siRNA-mouse. After 72 h, the cells were treated with TNF-α (3.0 ng ml −1 , e ) or IL-1 (3.0 ng ml −1 , f ) for the indicated times. The WCL was analysed by immunoblotting with the indicated antibodies. p47-m, p47-mouse. The depicted results are representative of three independent experiments. Full size image Ubiquitin-binding of p47 is crucial for IKK inhibition To elucidate the molecular mechanisms of p47-mediated IKK inhibition, we sought to determine the structural requirements for the inhibitory effect of p47 on IKK. p47 consists of three known domains: the N-terminal UBA domain (1–45) [45] , the central SEP (shp1, eyc and p47) domain (179–246) [39] and the C-terminal ubiquitin regulatory X (UBX) domain (286–370) [46] ( Fig. 4a ). p47 is crucial for the p97-mediated membrane fusion events that occur during the reassembly of the ER, the nuclear envelope and the Golgi apparatus [32] , [33] , [34] , [35] . As the ubiquitin-binding activity of p47 (via its UBA domain) and the association of p47 with p97 are essential for the p97-mediated reassembly of these organelles [32] , [37] , we first investigated whether similar conditions are required for p47-mediated IKK inhibition. To properly analyse the abilities of various p47 mutants to inhibit endogenous IKK, we silenced endogenous p47 before introducing expression vectors for p47 mutants, because p47 forms a trimer [32] , [39] . We constructed small interfering RNA (siRNA)-resistant p47 and the following p47 deletion mutants: ΔUBA (46–370) lacking the UBA domain, ΔUBX (1–246) lacking essential regions for p97 binding [47] , and ΔUBA/SEP (247–370) lacking the UBA and SEP domains and the linker sequence between them ( Fig. 4a ). The p47-knockdown cells were transfected with expression vectors encoding p47-WT or deletion mutants together with the NF-κB reporter. Both p47-WT and ΔUBX blocked NF-κB activation equally well ( Fig. 4b ), suggesting that the association of p47 with p97 is not essential for IKK inhibition. ΔUBA had a significantly reduced ability to inhibit NF-κB activation ( Fig. 4b ), indicating that the ubiquitin-binding activity of p47 is crucial for IKK inhibition. Interestingly, ΔUBA/SEP almost completely lacked the inhibitory effect ( Fig. 4b ), revealing that the sequence containing the SEP domain and linker region is also involved in IKK inhibition, albeit to a lesser extent than the UBA domain. To confirm the dispensability of p97, we examined the effect of p97 knockdown on the p47-mediated inhibition of NF-κB-driven reporter activity. p97 knockdown was successful because p97 was not detected, and the spliced form of XBP1 mRNA, an indication of ER stress, was observed [48] ( Fig. 4c ). p97 knockdown barely affected the p47-mediated inhibition of NF-κB-driven reporter activity ( Fig. 4c ), indicating that p97 is dispensable for the p47-mediated inhibition of NF-κB activation. 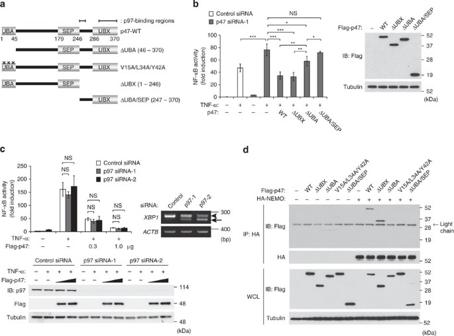Figure 4: The ubiquitin-binding activity of p47 is crucial for p47-mediated IKK inhibition. (a) A schematic representation of various mutants of p47. (b) HEK293T cells were transfected with control or p47 siRNA-1. After 24 h, the cells were transfected with plasmids encoding Flag-p47 or its various mutants together with a 3×κB-luc reporter. After 24 h, the cells were treated with TNF-α (1.0 ng ml−1) for 24 h, and the subsequent luciferase activity was measured. The results are given as the mean±s.d. (n=3). NS, not significant. Statistical significance was assessed using a Student'st-test. ***P<0.01, **P<0.02 and *,P<0.05. The expression levels of p47 and its various mutants were analysed. (c) HEK293T cells were transfected with control, p97 siRNA-1 or p97 siRNA-2. After 24 h, the cells were transfected with a 3×κB-luc reporter and Flag-p47 expression plasmid (0.3 or 1.0 μg). The cells were then treated with TNF-α (1.0 ng ml−1) for 24 h, and the subsequent luciferase activity was measured. The fold induction was calculated by dividing each luciferase activity measurement by that of the cells transfected with control siRNA without TNF-α stimulation. The results are given as the mean±s.d. (n=3). NS, not significant. Immunoblotting was performed using the WCL to confirm the silencing of p97 and expression levels of p47. RT–PCR was performed to detect unspliced (arrow head) and spliced (arrow)XBP1mRNA to confirm that the silencing of p97 induced ER stress. (d) HEK293T cells were transfected with expression plasmids encoding Flag-p47 or its various mutants (0.3 μg) together with a HA-NEMO expression plasmid (4 μg). After 24 h, the cell lysates were prepared and subjected to immunoprecipitation with an anti-HA antibody followed by immunoblotting with anti-Flag and anti-HA antibodies. The WCL was analysed by immunoblotting with anti-Flag and anti-tubulin antibodies. The depicted results are representative of three independent experiments. Consistent with the results shown in Figure 4b , p47-WT and ΔUBX bound similarly to NEMO, whereas the interaction of ΔUBA or ΔUBA/SEP with NEMO was barely observed ( Fig. 4d ). To further address the requirement for the ubiquitin-binding activity, we generated the V15A/L34A/Y42A mutant, wherein the three amino acid residues in the UBA domain that have been shown to form tight contacts with ubiquitin were substituted with alanines [39] , [49] ( Fig. 4a ). The V15A/L34A/Y42A mutant exhibited significantly reduced NEMO-binding activity ( Fig. 4d ). Taken together, both the p47/NEMO interaction and p47-mediated IKK inhibition require the ubiquitin-binding, but not the p97-binding activity of p47. Figure 4: The ubiquitin-binding activity of p47 is crucial for p47-mediated IKK inhibition. ( a ) A schematic representation of various mutants of p47. ( b ) HEK293T cells were transfected with control or p47 siRNA-1. After 24 h, the cells were transfected with plasmids encoding Flag-p47 or its various mutants together with a 3×κB-luc reporter. After 24 h, the cells were treated with TNF-α (1.0 ng ml −1 ) for 24 h, and the subsequent luciferase activity was measured. The results are given as the mean±s.d. ( n =3). NS, not significant. Statistical significance was assessed using a Student's t -test. *** P <0.01, ** P <0.02 and *, P <0.05. The expression levels of p47 and its various mutants were analysed. ( c ) HEK293T cells were transfected with control, p97 siRNA-1 or p97 siRNA-2. After 24 h, the cells were transfected with a 3×κB-luc reporter and Flag-p47 expression plasmid (0.3 or 1.0 μg). The cells were then treated with TNF-α (1.0 ng ml −1 ) for 24 h, and the subsequent luciferase activity was measured. The fold induction was calculated by dividing each luciferase activity measurement by that of the cells transfected with control siRNA without TNF-α stimulation. The results are given as the mean±s.d. ( n =3). NS, not significant. Immunoblotting was performed using the WCL to confirm the silencing of p97 and expression levels of p47. RT–PCR was performed to detect unspliced (arrow head) and spliced (arrow) XBP1 mRNA to confirm that the silencing of p97 induced ER stress. ( d ) HEK293T cells were transfected with expression plasmids encoding Flag-p47 or its various mutants (0.3 μg) together with a HA-NEMO expression plasmid (4 μg). After 24 h, the cell lysates were prepared and subjected to immunoprecipitation with an anti-HA antibody followed by immunoblotting with anti-Flag and anti-HA antibodies. The WCL was analysed by immunoblotting with anti-Flag and anti-tubulin antibodies. The depicted results are representative of three independent experiments. Full size image p47 binds to Lys63-linked and linear polyubiquitin chains NEMO becomes conjugated with either Lys63-linked or linear polyubiquitin chains upon stimulation [1] , [16] , [17] , [18] , [19] . Thus, we next determined which types of polyubiquitin linkages are recognized by p47. Purified recombinant wild-type or mutant His 6 -p47 protein bound to Ni-NTA resin ( Fig. 5a ) was mixed with various recombinant polyubiquitin chains, which were composed of di-ubiquitin and higher molecular weight species up to hepta-ubiquitin. p47 similarly bound to Lys48-linked tetra-ubiquitin, Lys63-linked tetra-ubiquitin, and linear tri- and tetra-ubiquitins ( Fig. 5b ). However, for polyubiquitin chains longer than tetra-ubiquitin, p47 preferentially bound to Lys63-linked and linear polyubiquitin chains than Lys48-linked polyubiquitin chains ( Fig. 5b ). Given that a large proportion of polyubiquitin chains in mammalian cells are likely to be longer than tetra-ubiquitin, these results suggest that p47 preferentially binds to Lys63-linked and linear polyubiquitin chains rather than Lys-48-linked polyubiquitin chains in vivo . The UBA domain is primarily involved in binding to all three types of polyubiquitin chains ( Fig. 5c–e ). The region composed of the SEP domain and linker region is also involved in binding to both Lys63-linked and linear polyubiquitin chains, although to a much lesser extent than the UBA domain ( Fig. 5c,d ). 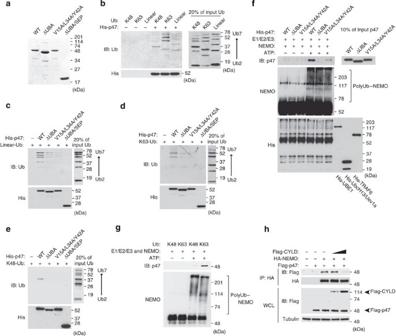Figure 5: The UBA domain of p47 preferentially interacts with Lys-63-linked and linear polyubiquitin chains. (a) The analysis of recombinant p47 and its mutant with 10% SDS–PAGE. (b) Ni-NTA resin-bound recombinant p47 or control resin was incubated with Lys48-linked, Lys63-linked, or linear polyubiquitin chains (Ub2~7). Polyubiquitin chains bound to p47 and a 20% input of polyubiquitin chains were analysed by immunoblotting with an anti-Ub antibody. (c–e) Recombinant p47 and various mutants that were bound to Ni-NTA resin were incubated with linear (c), Lys63-linked (d) or Lys48-linked polyubiquitin chains (e). (f) Recombinant His6-NEMO was incubated with recombinant His6-UBE1 (E1), His6-UbcH13/Uev1a (E2), His6-TRAF6 (E3) and ubiquitin in the presence or the absence of ATP. The reaction mixtures were then incubated with anti-NEMO antibody and protein G-sepharose. The immunoprecipitates were incubated with recombinant His6-p47 or its mutants, washed and analysed by immunoblotting with anti-p47, anti-NEMO and anti-His6antibodies. Ten percent of the inputs of p47 and its mutants were analysed by immunoblotting with an anti-p47 antibody. (g) Recombinant His6-NEMO was incubated with UBE1 (E1), UbcH5c (E2), His6-cIAP1 (E3), and ubiquitin containing only lysine 48 (K48) or only lysine 63 (K63) in the presence or the absence of ATP. The reaction mixtures were incubated with an anti-NEMO antibody and protein G-sepharose. The immunoprecipitates were incubated with recombinant His6-p47, washed and analysed by immunoblotting with anti-p47 and anti-NEMO antibodies. (h) HEK293T cells were transfected with expression plasmids encoding HA-NEMO (1.0 μg) and Flag-p47 (0.3 μg) in combination with the expression plasmid for Flag-CYLD (0.3, 3.0 μg). After 48 h, the cell lysates were subjected to immunoprecipitation with an anti-HA antibody followed by immunoblotting with anti-Flag and anti-HA antibodies. The WCL was analysed by immunoblotting with anti-Flag and anti-tubulin antibodies. The depicted results are representative of three independent experiments. Figure 5: The UBA domain of p47 preferentially interacts with Lys-63-linked and linear polyubiquitin chains. ( a ) The analysis of recombinant p47 and its mutant with 10% SDS–PAGE. ( b ) Ni-NTA resin-bound recombinant p47 or control resin was incubated with Lys48-linked, Lys63-linked, or linear polyubiquitin chains (Ub 2~7 ). Polyubiquitin chains bound to p47 and a 20% input of polyubiquitin chains were analysed by immunoblotting with an anti-Ub antibody. ( c – e ) Recombinant p47 and various mutants that were bound to Ni-NTA resin were incubated with linear ( c ), Lys63-linked ( d ) or Lys48-linked polyubiquitin chains ( e ). ( f ) Recombinant His 6 -NEMO was incubated with recombinant His 6 -UBE1 (E1), His 6 -UbcH13/Uev1a (E2), His 6 -TRAF6 (E3) and ubiquitin in the presence or the absence of ATP. The reaction mixtures were then incubated with anti-NEMO antibody and protein G-sepharose. The immunoprecipitates were incubated with recombinant His 6 -p47 or its mutants, washed and analysed by immunoblotting with anti-p47, anti-NEMO and anti-His 6 antibodies. Ten percent of the inputs of p47 and its mutants were analysed by immunoblotting with an anti-p47 antibody. ( g ) Recombinant His 6 -NEMO was incubated with UBE1 (E1), UbcH5c (E2), His 6 -cIAP1 (E3), and ubiquitin containing only lysine 48 (K48) or only lysine 63 (K63) in the presence or the absence of ATP. The reaction mixtures were incubated with an anti-NEMO antibody and protein G-sepharose. The immunoprecipitates were incubated with recombinant His 6 -p47, washed and analysed by immunoblotting with anti-p47 and anti-NEMO antibodies. ( h ) HEK293T cells were transfected with expression plasmids encoding HA-NEMO (1.0 μg) and Flag-p47 (0.3 μg) in combination with the expression plasmid for Flag-CYLD (0.3, 3.0 μg). After 48 h, the cell lysates were subjected to immunoprecipitation with an anti-HA antibody followed by immunoblotting with anti-Flag and anti-HA antibodies. The WCL was analysed by immunoblotting with anti-Flag and anti-tubulin antibodies. The depicted results are representative of three independent experiments. Full size image To confirm that the binding of p47 to NEMO is mediated by the polyubiquitin chains conjugated to NEMO, recombinant His 6 -NEMO was incubated with His 6 -UBE1 (E1), His 6 -Ubc13/Uev1 (E2), His 6 -TRAF6 (E3) and ATP to catalyse the Lys63-linked polyubiquitination of NEMO. As a control experiment, the same reaction was carried out without ATP. The immunocomplexes precipitated by an anti-NEMO antibody were incubated with recombinant wild-type or mutant p47 and subjected to immunoblotting. As the extent of NEMO ubiquitination was similar in the reactions with ATP and as comparable amounts of NEMO and other proteins (except p47) co-precipitated in all of the reactions ( Fig. 5f ), wild-type or mutant p47 bound to NEMO could be measured by immunoblotting, using the anti-p47 antibody. p47 was observed to bind to NEMO only when NEMO was conjugated to Lys63-linked polyubiquitin chains, and this interaction required the ubiquitin-binding activity of p47 ( Fig. 5f ). To further confirm the linkage-type specificity, recombinant His 6 -NEMO was subjected to in vitro ubiquitination using cIAP1 as an E3 enzyme, with ubiquitin containing only Lys-48 or only Lys-63 to generate NEMO with Lys48-linked or Lys63-linked polyubiquitin chains [14] , [50] . p47 bound to NEMO with Lys63-linked polyubiquitin chains, but not to NEMO with Lys48-linked chains ( Fig. 5g ). Moreover, p47 failed to bind to NEMO in the presence of CYLD ( Fig. 5h ). Taken together, these results indicate that p47 does not bind to the non-ubiquitinated form of NEMO, but does bind to NEMO conjugated with Lys63-linked or linear polyubiquitin chains. p47 post-translationally controls NEMO protein levels Given that p47 binds to polyubiquitinated NEMO, we hypothesized that p47 may induce the degradation of polyubiquitinated NEMO, because p47 is involved in the degradation of polyubiquitinated proteins [38] . Each of the components of the IKK complex, including IKKα, IKKβ, NEMO and Hsp90, was expressed in HEK293T cells with or without p47. Whereas the expression levels of IKKα, IKKβ and Hsp90 were not affected ( Fig. 6a ), NEMO expression was decreased by co-expression of p47 in a dose-dependent manner ( Fig. 6b ). As the promoters that drive NEMO and Hsp90 expression were the same, the reduction in NEMO expression could not be due to transcriptional squelching. p47 knockdown resulted in enhanced HA-NEMO expression derived from the transfected plasmid, whereas complementation with Flag-p47 resulted in decreased HA-NEMO expression ( Fig. 6c ). The expression level of HA-IKKβ derived from the co-transfected plasmid was not affected by p47 knockdown or subsequent complementation thereof ( Fig. 6c ). As NEMO is an integral component of the IKK complex, we next addressed whether p47 degrades IKKβ-associated NEMO. HEK293T cells were co-transfected with expression plasmids for NEMO, HA-IKKβ and Flag-p47. Immunoprecipitation of IKKβ revealed that p47 degraded IKKβ-associated NEMO ( Fig. 6d ). NEMO expression, but not IKKβ expression, was significantly reduced even when they were co-expressed ( Fig. 6d ). In addition, the overexpression of p47 resulted in a reduction of endogenous NEMO after, but not before, TNF-α stimulation, although the extent of the endogenous NEMO reduction was less significant than that of overexpressed NEMO ( Fig. 6e ). These results strongly suggest that p47 selectively degrades NEMO and leaves IKKα/β intact upon stimulation. p97 knockdown barely affected the p47-mediated reduction of NEMO ( Fig. 6f ). The ubiquitin-binding activity of p47 was crucial for the p47-mediated reduction of NEMO, and the sequence containing the SEP domain and the linker region was also involved, albeit to a lesser extent when compared with the UBA domain ( Fig. 6g ). Furthermore, CYLD inhibited the p47-mediated reduction of NEMO in a dose-dependent manner ( Fig. 6h ), indicating that the ubiquitinated form of NEMO is required for the p47-mediated NEMO reduction. However, the non-ubiquitinated form of NEMO was also reduced in the presence of ubiquitinated NEMO ( Fig. 6b ), suggesting that the non-ubiquitinated and ubiquitinated forms of NEMO associate with each other and that p47 targets the non-ubiquitinated form of NEMO via ubiquitinated NEMO. As TRAF6 and NEMO become conjugated with Lys63-linked polyubiquitin chains upon stimulation [2] , [7] , we next addressed whether p47 overexpression results in a reduction of TRAF6. HEK293T cells were transfected with an expression plasmid for Flag-NEMO or Flag-TRAF6 in combination with increasing amounts of the Flag-p47 expression plasmid. NEMO expression was reduced by co-expression with p47 even when the lowest amount of the p47 expression plasmid (0.1 μg) was transfected. In contrast, TRAF6 expression was reduced only when the highest amount of the p47 expression plasmid (1.0 μg) was transfected ( Fig. 6i ). These results suggest that p47 may recognize polyubiquitinated NEMO more efficiently than polyubiquitinated TRAF6. Therefore, p47 is likely to recognize NEMO itself in addition to the polyubiquitin chain conjugated to NEMO. Given that p47 does not bind to non-ubiquitinated NEMO ( Fig. 5f,h ), the polyubiquitination of NEMO may induce a structural change of NEMO to enable p47 to recognize NEMO itself. 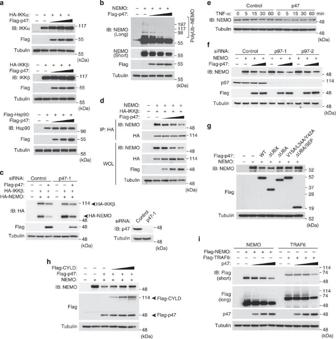Figure 6: p47 reduces NEMO protein expression. (a) HEK293T cells were transfected with an HA-IKKα, HA-IKKβ, or Flag-Hsp90 expression plasmid (0.1 μg) together with a Flag-p47 expression plasmid (0.1, 0.3 or 1 μg). (b) HEK293T cells were transfected with a NEMO expression plasmid (0.1 μg) together with a Flag-p47 expression plasmid (0.1, 0.3 or 1 μg). (c) HEK293T cells were transfected with control or p47 siRNA. After 24 h, the cells were transfected with a control or Flag-p47 expression plasmid (1.0 μg) followed by transfection with HA-NEMO and HA-IKKβ expression plasmids (0.5 μg). (d) HEK293T cells were transfected with expression plasmids encoding NEMO (0.1 μg), HA-IKKβ (0.1 μg) and Flag-p47 (0.1, 0.3 or 1.0 μg). After 48 h, cell lysates were subjected to immunoprecipitation with an anti-HA antibody. (e) HEK293T cells were transfected with a control or Flag-p47 expression plasmid. After 48 h, cells were treated with TNF-α (10 ng ml−1). (f) HEK293T cells were transfected with control or p97 siRNA. After 24 h, the cells were transfected with NEMO (0.1 μg) and Flag-p47 (0.3 or 1.0 μg) expression plasmids. (g) HEK293T cells were transfected with the NEMO expression plasmid (0.1 μg) together with the expression plasmid for Flag-p47 or its various mutants (1 μg). (h) HEK293T cells were transfected with expression plasmids encoding NEMO (0.1 μg), Flag-p47 (1.0 μg) and Flag-CYLD (0.1, 0.3 or 1.0 μg). (i) HEK293T cells were transfected with 0.1 μg of a pRK5-Flag-NEMO or pRK5-Flag-TRAF6 expression plasmid together with a p47 expression plasmid (0.1, 0.3 or 1.0 μg). After 48 h, the WCL was analysed. The depicted results are representative of three independent experiments. Figure 6: p47 reduces NEMO protein expression. ( a ) HEK293T cells were transfected with an HA-IKKα, HA-IKKβ, or Flag-Hsp90 expression plasmid (0.1 μg) together with a Flag-p47 expression plasmid (0.1, 0.3 or 1 μg). ( b ) HEK293T cells were transfected with a NEMO expression plasmid (0.1 μg) together with a Flag-p47 expression plasmid (0.1, 0.3 or 1 μg). ( c ) HEK293T cells were transfected with control or p47 siRNA. After 24 h, the cells were transfected with a control or Flag-p47 expression plasmid (1.0 μg) followed by transfection with HA-NEMO and HA-IKKβ expression plasmids (0.5 μg). ( d ) HEK293T cells were transfected with expression plasmids encoding NEMO (0.1 μg), HA-IKKβ (0.1 μg) and Flag-p47 (0.1, 0.3 or 1.0 μg). After 48 h, cell lysates were subjected to immunoprecipitation with an anti-HA antibody. ( e ) HEK293T cells were transfected with a control or Flag-p47 expression plasmid. After 48 h, cells were treated with TNF-α (10 ng ml −1 ). ( f ) HEK293T cells were transfected with control or p97 siRNA. After 24 h, the cells were transfected with NEMO (0.1 μg) and Flag-p47 (0.3 or 1.0 μg) expression plasmids. ( g ) HEK293T cells were transfected with the NEMO expression plasmid (0.1 μg) together with the expression plasmid for Flag-p47 or its various mutants (1 μg). ( h ) HEK293T cells were transfected with expression plasmids encoding NEMO (0.1 μg), Flag-p47 (1.0 μg) and Flag-CYLD (0.1, 0.3 or 1.0 μg). ( i ) HEK293T cells were transfected with 0.1 μg of a pRK5-Flag-NEMO or pRK5-Flag-TRAF6 expression plasmid together with a p47 expression plasmid (0.1, 0.3 or 1.0 μg). After 48 h, the WCL was analysed. The depicted results are representative of three independent experiments. Full size image p47 targets ubiquitinated NEMO for lysosomal degradation To support the hypothesis that p47 induces the degradation of NEMO, p47 and NEMO were co-expressed in HEK293T cells, and the cells were treated with MG132 (a proteasome inhibitor) or E64D in combination with pepstatin A (lysosome inhibitors). NEMO expression was significantly restored in response to treatment with E64D/pepstatin A, but not with MG132 ( Fig. 7a ), suggesting that p47 induces the lysosomal degradation of polyubiquitinated NEMO. To further confirm the degradation of NEMO under physiological conditions, the TNF-α-induced polyubiquitination of endogenous NEMO was analysed. The enhanced accumulation of polyubiquitinated NEMO was observed in p47-knockdown cells ( Fig. 7b ) and in the E64D/pepstatin A-treated cells, but not in the MG132-treated cells ( Fig. 7c ). Similar results were obtained using a different experimental protocol ( Supplementary Fig. S4 ) and with other lysosome inhibitors such as chloroquine and bafilomycin A1 ( Supplementary Fig. S5 ). To demonstrate that NEMO is recruited to the lysosome after TNF-α stimulation, HeLa cells were treated with chloroquine followed by treatment with TNF-α, and the subcellular localization of NEMO and lysosomal-associated membrane protein 1 (LAMP-1), a late endosomal–lysosomal marker, was analysed using confocal immunofluorescence microscopy. A small proportion of NEMO colocalized with LAMP-1 in the lysosome in a TNF-α-stimulation-dependent manner ( Fig. 7d ). Moreover, chloroquine treatment enhanced TNF-α-induced NF-κB-dependent transcription ( Fig. 7e ) and interaction of p47 with NEMO ( Fig. 7f ). Collectively, these results strongly suggest that p47 targets polyubiquitinated NEMO for lysosomal degradation, thereby negatively regulating NF-κB activation. 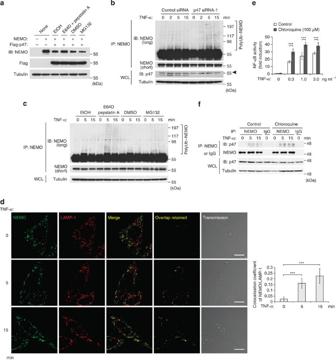Figure 7: p47 induces the lysosomal degradation of polyubiquitinated NEMO. (a) HEK293T cells were transfected with NEMO (0.1 μg) and Flag-p47 (1 μg) expression plasmids. The cells were treated with E64D (5 μg ml−1)/pepstatin A (1 μg ml−1) for 12 h or treated with MG132 (10 μM) for 2 h. (b) HeLa cells were transfected with control or p47 siRNA. After TNF-α (10 ng ml−1) stimulation, the cell lysates were subjected to immunoprecipitation with an anti-NEMO antibody followed by immunoblotting with an anti-NEMO antibody. An arrowhead denotes non-specific bands. (c) HeLa cells were treated with E64D/pepstatin A for 2 h or with MG132 for 2 h. After TNF-α stimulation, cell lysates were subjected to immunoprecipitation as described inb. (d) HeLa cells were treated with chloroquine (100 μM) for 2 h. After TNF-α stimulation, the subcellular localization of NEMO and LAMP-1 was analysed using confocal immunofluorescence microscopy. The Manders' colocalization coefficients of NEMO/LAMP-1 were analysed by Olympus imaging software. The results are given as the mean±s.d. (n=30) and are representative of three independent experiments. Scale bar, 10 μm. (e) HEK293T cells were transfected with a 3×κB-luc. After 36 h, the cells were untreated or treated with chloroquine for 2 h. After 8 h of TNF-α stimulation, the luciferase activity was measured. The fold induction was calculated by dividing each luciferase activity by that of the control without TNF-α stimulation. The results are given as the mean±s.d. (n=3). (f) HeLa cells were treated with chloroquine for 2 h and then stimulated with TNF-α. The cell lysates were subjected to immunoprecipitation with a control IgG or anti-NEMO antibody. The depicted results are representative of three independent experiments. Statistical significance was assessed using a Student'st-test. ***P<0.01. Figure 7: p47 induces the lysosomal degradation of polyubiquitinated NEMO. ( a ) HEK293T cells were transfected with NEMO (0.1 μg) and Flag-p47 (1 μg) expression plasmids. The cells were treated with E64D (5 μg ml −1 )/pepstatin A (1 μg ml −1 ) for 12 h or treated with MG132 (10 μM) for 2 h. ( b ) HeLa cells were transfected with control or p47 siRNA. After TNF-α (10 ng ml −1 ) stimulation, the cell lysates were subjected to immunoprecipitation with an anti-NEMO antibody followed by immunoblotting with an anti-NEMO antibody. An arrowhead denotes non-specific bands. ( c ) HeLa cells were treated with E64D/pepstatin A for 2 h or with MG132 for 2 h. After TNF-α stimulation, cell lysates were subjected to immunoprecipitation as described in b . ( d ) HeLa cells were treated with chloroquine (100 μM) for 2 h. After TNF-α stimulation, the subcellular localization of NEMO and LAMP-1 was analysed using confocal immunofluorescence microscopy. The Manders' colocalization coefficients of NEMO/LAMP-1 were analysed by Olympus imaging software. The results are given as the mean±s.d. ( n =30) and are representative of three independent experiments. Scale bar, 10 μm. ( e ) HEK293T cells were transfected with a 3×κB-luc. After 36 h, the cells were untreated or treated with chloroquine for 2 h. After 8 h of TNF-α stimulation, the luciferase activity was measured. The fold induction was calculated by dividing each luciferase activity by that of the control without TNF-α stimulation. The results are given as the mean±s.d. ( n =3). ( f ) HeLa cells were treated with chloroquine for 2 h and then stimulated with TNF-α. The cell lysates were subjected to immunoprecipitation with a control IgG or anti-NEMO antibody. The depicted results are representative of three independent experiments. Statistical significance was assessed using a Student's t -test. *** P <0.01. Full size image Potential involvement of p47 in cancer development Analysis of the Oncomine database [51] revealed that p47 expression is downregulated in some human cancers, including prostate carcinoma, glioblastoma and breast carcinoma. In addition, analysis of Gene Expression Omnibus data [52] revealed significant reduction of p47 expression in acute and chronic adult T-cell leukaemia (ATL; Supplementary Fig. S6a ), in which the constitutive activation of NF-κB mediated by Tax-dependent and independent mechanisms is crucial in leukemogenesis and survival of tumour cells [53] . On the basis of our preliminary experiments, when compared with non-infected Jurkat T-cell line, p47 expression is significantly reduced at both the mRNA and protein levels in ATL patient-derived and human T-cell leukaemia virus-1-infected cell lines, in which various NF-κB target genes were highly expressed due to constitutive NF-κB activation ( Supplementary Fig. S6b,c ). Moreover, Tax inhibited the interaction between p47 and the IKK complex, whereas enhanced p47 expression inhibited NF-κB activation in Tax-expressing cells ( Supplementary Fig. S6d, e ), suggesting that reduced p47 expression may be involved in leukemogenesis. Thus, the altered expression or function of p47 in vivo may result in constitutive NF-κB activation, which may trigger development of various cancers. Excess and/or prolonged NF-κB activation leads to the development of inflammatory diseases, autoimmunity and cancer [23] , [24] , [25] , [26] . However, it is not fully understood how the amplitude and duration of NF-κB activation are tightly regulated. p47 has previously been identified as an essential factor for the membrane reassembly of the ER, the nuclear envelope and the Golgi apparatus [32] , [33] , [34] , [35] . Here we demonstrate that p47 associates with the IKK complex via NEMO within 5 min of stimulation with TNF-α or IL-1. Importantly, the association of p47 with the IKK complex inhibits the stimulation-induced activation of this complex, thereby inhibiting the expression of NF-κB target genes. Thus, p47 is crucial for maintaining appropriate expression levels of cytokines and chemokines, which mediate inflammation. Several lines of evidence indicate that the negative regulation of IKK by p47 is triggered by the binding of p47 to Lys63-linked or linear polyubiquitin chains that are conjugated to NEMO. First, the inactivation of the UBA domain significantly impairs the p47-mediated inhibition of NF-κB activation. Second, p47 binds to Lys63-linked and linear polyubiquitin chains primarily through its UBA domain. In addition, the binding of p47 to NEMO depends on its UBA domain and polyubiquitin. The co-expression of NEMO with p47 resulted in the degradation of NEMO but not of IKKβ associated with NEMO. This degradation required the UBA domain of p47 and lysosomal proteases but did not require the proteasome. We did not observe a stimulation-dependent degradation of endogenous NEMO, likely because only a small amount of endogenous NEMO is ubiquitinated. However, we did detect a significant level of ubiquitinated NEMO when NEMO was overexpressed. An enhanced TNF-α-induced accumulation of polyubiquitinated endogenous NEMO was observed when p47 was silenced or when cells were treated with lysosomal inhibitors but not with proteasome inhibitors. Moreover, a small but significant portion of NEMO was transferred to the lysosome upon TNF-α stimulation. Given that Shp1, a yeast homologue of p47, binds Atg8, a yeast homologue of LC3 that is required for the elongation of the nascent autophagosome [54] , our results suggest that p47 deprives the activated IKK complex of ubiquitinated NEMO and targets ubiquitinated NEMO for lysosomal degradation ( Fig. 8 ). In this sense, p47 is similar to p62 and NBR1, which also each have a UBA domain and target ubiquitinated protein aggregates to autophagosomes via their interaction with LC3 (refs [55] , [56] ). However, involvement of autophagic clearance in the p47-mediated NEMO degradation remains to be elucidated. 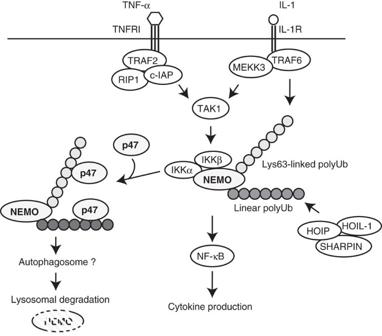Figure 8: A model illustrating p47-mediated IKK inhibition. Upon TNF-α and IL-1 stimulation, TRAF6 catalyses the conjugation of Lys63-linked polyubiquitin chains to NEMO, and LUBAC (linear ubiquitin chain assembly complex), which is composed of HOIP, HOIL-1 and SHARPIN, catalyses the conjugation of linear polyubiquitin chains to NEMO. p47 binds to polyubiquitinated NEMO and induces the degradation of NEMO through a lysosome-dependent pathway. Involvement of autophagy in the NEMO degradation remains to be elucidated. PolyUb, polyubiquitin chain. Figure 8: A model illustrating p47-mediated IKK inhibition. Upon TNF-α and IL-1 stimulation, TRAF6 catalyses the conjugation of Lys63-linked polyubiquitin chains to NEMO, and LUBAC (linear ubiquitin chain assembly complex), which is composed of HOIP, HOIL-1 and SHARPIN, catalyses the conjugation of linear polyubiquitin chains to NEMO. p47 binds to polyubiquitinated NEMO and induces the degradation of NEMO through a lysosome-dependent pathway. Involvement of autophagy in the NEMO degradation remains to be elucidated. PolyUb, polyubiquitin chain. Full size image p47 preferentially binds to Lys63-linked and linear polyubiquitin chains versus Lys48-linked polyubiquitin chains when they contain five or more ubiquitin moieties. As previous studies have shown that the p47 UBA domain binds monoubiquitin [37] , [39] , implying that the native p47 homotrimer should bind three ubiquitin units, the relative positions and orientations of the three UBA domains in the p47 trimer may account for the linkage and length specificities of the p47–polyubiquitin interaction. Interestingly, we found that the sequence containing the SEP domain and the linker region also contribute to ubiquitin binding and IKK inhibition. As the SEP and UBX domains are involved in p47 trimer formation [39] , the trimerization of the linker plus the SEP region may result in the formation of a lower-affinity ubiquitin-binding surface that cooperates with the UBA domain to increase the overall polyubiquitin chain affinity. The association of p47 with the cytosolic AAA ATPase p97 is crucial for the membrane reassembly of organelles [32] ; however, p97 is dispensable for p47-mediated IKK inhibition, suggesting that cytosolic p47 associates with distinct partner proteins, such as LC3 or proteins required for targeting p47 to the autophagosome. The identification of p47-associated proteins in the cytosol is essential for understanding how p47 induces the lysosomal degradation of polyubiquitinated NEMO. DUBs, such as A20 and CYLD, have pivotal roles in the negative regulation of NF-κB activation [27] , [28] , [29] , [30] . CYLD is a tumour suppressor protein whose inactivation results in familial cylindromatosis [25] . In contrast, A20-deficient mice develop severe inflammation and cachexia [31] . Although p47 and these DUBs recognize polyubiquitin chains that are generated for NF-κB activation, p47 negatively regulates IKK activation in a manner that is mechanistically distinct from that of A20 and CYLD. It has been proposed that A20 regulates both the initial and termination phases of stimulation-induced NF-κB activation [57] , [58] , [59] , whereas CYLD is involved in blocking spontaneous NF-κB activation as well as in the initial phase [25] , [60] . Given that p47 and these DUBs negatively regulate the initial phase of stimulation-induced NF-κB activation and that CYLD inhibits the interaction of p47 with NEMO, p47 and these two DUBs could co-operatively regulate the initial phase of stimulation-induced NF-κB activation for achieving the appropriate expression levels of NF-κB target genes. Consistent with this idea, significant reduction of p47 expression was observed in ATL cells, which show high levels of constitutive NF-κB activation that protects ATL cells from apoptosis [53] . A better understanding of the mechanisms of p47-mediated IKK inhibition should eventually lead to the development of novel therapeutic approaches that promote the activity of p47. Plasmids Human cDNAs encoding Hsp90, p47 and CYLD were generated by PCR and inserted into the pRK5 vector. The NEMO cDNA was obtained from S Yamaoka (Tokyo Medical and Dental University) and inserted into the pcDNA3 vector (Life Technologies, Carlsbad, CA, USA) or into the pRK5 vector. pRcβact-3HA-IKKα and -IKKβ were obtained from M. Karin (University of California); 3×κB-luc was obtained from S Miyamoto (University of Wisconsin). Antibodies and reagents Antibodies used were as follows: anti-p-IκBα (9246), anti-IκBα (9242), anti-p-JNK (9251), anti-p-p38 (9211), anti-p-ERK (9101), anti-IKKα (2682), anti-IKKβ (2684) and anti-NEMO (2695) (Cell Signaling Technology, Danvers, MA, USA); anti-p65 (sc-8008), anti-GST (sc-459), anti-HA-tag (sc-805), anti-CYLD (sc-744435) and anti-ubiquitin (sc-8017) (Santa Cruz Biotechnology, Santa Cruz, USA); anti-Flag M2 (F3165) (Sigma, St Louis, MO, USA); anti-tubulin (CP06) (Millipore, Darmstadt, Germany); anti-p47 (H00055968-B01P) (Abnova, Taipei City, Taiwan); anti-A20 (60-6629-81) (eBioscience, San Diego, CA, USA); anti-p97 (612182) (BD Transduction Laboratories, Franklin Lakes, NJ, USA); and anti-His-tag (PM032) (MBL, Nagoya, Japan). All antibodies were used at a 2,000-fold dilution. Reagents used were as follows: MG132, E64D, and pepstatin A (Peptide Institute, Osaka, Japan) and chloroquine (Wako, Osaka, Japan). Cell culture and transfection A20 −/− MEF was obtained from A. Ma (University of California). Cyld − /− MEF was obtained from S. -C. Sun (University of Texas). HEK293T, HeLa and MEF cells were maintained in DMEM supplemented with 10% fetal bovine serum (FBS). Jurkat cells were maintained in RPMI1640 with 10% FBS. Sf9 cells were maintained in Sf900 IIISFM (Life Technologies) supplemented with 10% FBS. The DNA transfection was performed via the calcium phosphate method. siRNAs were transfected using RNAiMAX reagents (Life Technologies). Control siRNA and the following double-stranded siRNAs (Life Technologies) were used: p47-1 sense/anti-sense, 5′-CAACGAGCUGGUGGAUGAUCUCUUU-3′/5′-AAAGAGAUCAUCCACCAGCUCGUUG-3′; p47-2 sense/anti-sense, 5′-GAGAGACCAGUAAACCGAGACCAUU-3′/5′-AAUGGUCUCGGUUUACUGGUCUCUC-3′; p47-mouse sense/anti-sense, 5′-UGACAUCCUUCAGAGACCUCAUUCA-3′/5′-UGAAUGAGGUCUCUGAAGGAUGUCA-3′; p97-1 sense/anti-sense, 5′-CCCAAGAUGGAUGAAUUGCAGUUGU-3′/5′-ACAACUGCAAUUCAUCCAUCUUGGG-3′; p97-2 sense/anti-sense, 5′-GGAGUUCAAAGUGGUGGAAACAGAU-3′/5′-AUCUGUUUCCACCACUUUGAACUCC-3′. Mass spectrometry Jurkat cells expressing Flag-NEMO were suspended in hypotonic buffer (10 mM Tris–HCl at pH 7.4, 1.5 mM MgCl 2 , 10 mM KCl, 0.5 mM dithiothreitol (DTT) and protease inhibitor cocktail (Roche, Basel, Switzerland)), and then lysed with a Dounce homogenizer. Cell debris was removed by ultracentrifugation at 100,000 g for 1 h to prepare the S-100 cytosolic fraction. Recombinant Tax protein was added to the S-100 fraction, and the resultant reaction mixture was incubated at 30 °C for 1 h. Protein complexes containing NEMO were then immunoprecipitated using an anti-Flag antibody and were eluted with Flag peptides. The eluted proteins were digested with trypsin and loaded onto an automated nanoflow liquid chromatography system (Dina; KYA Technologies, Tokyo, Japan) coupled to a quadrupole time-of-flight tandem mass spectrometer (Q-Star Elite; AB SCIEX, Framingham, MA, USA). The tandem mass spectrometry signals were processed against human protein sequences in the NCBI RefSeq database using the Mascot algorithm (Matrix Science, Boston, MA, USA). Immunoprecipitation and immunoblot analysis For immunoprecipitation, cells were lysed in TNE buffer (20 mM Tris–HCl at pH 7.5, 150 mM NaCl, 2 mM EDTA, 1 mM MgCl 2 , 10 mM NaF, 1% (v/v) NP-40, 10 mM β-glycerophosphate, 1 mM Na 3 VO 4 , 1 mM DTT, 5 mM N -ethylmaleimide, protease inhibitor cocktail) and centrifuged at 22,000 g for 15 min at 4 °C to remove the insoluble fraction. The supernatants were incubated with 0.5 μg of antibody plus 10 μl of protein G-sepharose (GE Healthcare, Piscataway, NJ, USA). The immunoprecipitates were washed three times and subjected to immunoblotting. For immunoblot analysis, immunoprecipitates or whole-cell lysates were separated by SDS–PAGE and transferred to polyvinylidenedifluoride membranes (Immobilon P, Millipore). The membranes were then incubated with the primary antibodies. Immunoreactive proteins were visualized with anti-rabbit or anti-mouse IgG conjugated to horseradish peroxidase (GE Healthcare) followed by processing with an ECL detection system (GE Healthcare). Luciferase reporter assay HEK293T cells were transfected with the plasmids encoding wild type or various p47 mutants together with 20 ng of luciferase reporter (3×κB-luc) and 30 ng of β-actin–β-galactosidase plasmid. After 24 h of incubation, the cells were treated with TNF-α for 24 h, and the luciferase activity was measured using the Luciferase Assay System (Toyo Ink, Tokyo, Japan). β-galactosidase activity was used to normalize the transfection efficiency. In some experiments, siRNAs were transfected 24 h before plasmid transfection. In vitro IKK kinase assay HEK293T cells were treated with TNF-α (10 ng ml −1 ) for the indicated times and lysed in TNE buffer without N -ethylmaleimide. IKK complexes were immunoprecipitated with an anti-NEMO antibody. The immunoprecipitates were incubated at 30 °C for 1 h in kinase buffer (50 mM Tris–HCl at pH 7.5, 5 mM MgCl 2 , 2 mM ATP, 10 mM creatine phosphate, 3.5 U ml −1 creatine kinase, 5 mM NaF, 20 mM β-glycerophosphate and 1 mM Na 3 VO 4 ) with 100 ng of GST-IκBα (amino acids 1–54). The reaction mixtures were subjected to immunoblotting using an anti-p-IκBα antibody, and the intensities of the bands were quantified using ImageJ software (National Institutes of Health). Electrophoretic mobility shift assay HeLa cells were stimulated with TNF-α or IL-1 and then suspended in hypotonic buffer. The cell suspensions were incubated on ice for 30 min and centrifuged at 22,000 g for 5 min at 4 °C. The nuclear pellets were suspended in extraction buffer (20 mM HEPES at pH 7.9, 420 mM NaCl, 1.5 mM MgCl 2 , 0.2 mM EDTA, 0.5 mM DTT, 25% (v/v) glycerol and a protease inhibitor cocktail) and incubated on ice for 20 min. The nuclear extracts were obtained from the supernatants. The nuclear extracts (3 μg) were incubated with 32 P-labelled oligonucleotides that contained the NF-κB-binding site or the Oct-1-binding site for 25 min at 25 °C. The DNA–protein complexes were separated by electrophoresis with a 4% polyacrylamide gel. The following oligonucleotides were used: NF-κB, 5′-AGCTTCAGAGGGGACTTTCCGAGAGG-3′, and 5′-TCGACCTCTCGGAAAGTCCCCTCTGA-3′; and Oct-1, 5′-TGTCGAATGCAAATCACTAGAA-3′ and 5′-TGTTCTAGTGATTTGCATTCGA-3′. Quantitative real-time reverse transcriptase PCR assays The total RNA was isolated from TNF-α- or IL-1-treated HeLa cells with Trizol reagent (Life Technologies). cDNA was synthesized from 1 μg of total RNA with Prime Script II (Takara Bio, Shiga, Japan). Quantitative real-time PCR analysis was performed on a 7300 Fast Real-Time PCR System (Life Technologies) using FastStart Universal SYBR Green Master (Roche). The level of β-actin expression was used to normalize the data. The following primers were used: IL-8 sense/anti-sense, 5′-ATGACTTCCAAGCTGGCCGT-3′/5′-TTACATAATTTCTGTGTTGGC-3′; TNF-α sense/anti-sense, 5′-GGAGAAGGGTGACCGACTCA-3′/5′-TGCCCAGACTCGGCAAAG-3′; β-actin sense/anti-sense, 5′-TTCTACAATGAGCTGCGTGTG-3′/5′-CCTTAATGTCACGCACGATTT-3′. Recombinant proteins His 6 -tagged p47, NEMO, TRAF6, cIAP1 and Tax were produced using the Bac-to-Bac Baculovirus Expression System (Life Technologies). Briefly, a 50-ml culture of Sf9 cells (1×10 6 cells ml −1 ) was infected with recombinant baculovirus expressing each protein. Seventy-two hours after infection, cells were harvested, and His 6 -tagged recombinant proteins were purified using Ni-NTA resin (QIAGEN, Valencia, CA, USA). His 6 -UBE1, His 6 -UbcH13/Uev1a, UbcH5c, and ubiquitin (wild-type, K63 only, K48 only) were purchased (Boston Biochem, Cambridge, MA, USA). In vitro binding assays of p47 and polyubiquitinated NEMO In Figure 5f , the reactions were performed at 37 °C for 2 h in 50 μl of kinase buffer containing 1 μg of His 6 -UBE1, 2 μg of His 6 -UbcH13/Uev1a, 2 μg of His 6 -TRAF6, 1 μg of His 6 -NEMO and 50 μg of ubiquitin. In Figure 5g , the reactions were performed at 37 °C for 2 h in 25 μl of kinase buffer containing 0.5 μg of UBE1, 0.85 μg of UbcH5c, 0.2 μg of His 6 -cIAP1, 0.5 μg of His 6 -NEMO and 5 μg of ubiquitin containing only Lys-48 or only Lys-63. After incubation, the reaction mixtures were incubated with 1 μg of an anti-NEMO antibody together with 10 μl of protein G-sepharose. The immunoprecipitates were incubated with recombinant His 6 -p47 or its mutants at 4 °C for 2 h. After washing, His 6 -p47 or its mutants bound to the immunoprecipitates were analysed by immunoblotting. In vitro binding assays of p47 and polyubiquitin chains Ni-NTA resin was incubated with 10 μg of p47 and its mutants at 4 °C for 2 h in binding buffer (20 mM Tris–HCl at pH 7.5, 150 mM NaCl, 0.5% (v/v) NP-40, 2.5 mg ml −1 BSA, 20 mM imidazole and 5 mM 2-mercaptoethanol). The beads were then incubated with 1.0 μg of linear (Enzo Lifescience, Farmingdale, NY, USA), Lys63-, or Lys48-linked polyubiquitin chains (Boston Biochem) at 4 °C for 2 h. After incubation, the beads were washed and subjected to immunoblotting. Immunofluorescence HeLa cells were treated with chloroquine (100 μM) for 2 h. After TNF-α stimulation, the cells were washed with PBS and fixed in 4% paraformaldehyde followed by permeabilization with 1% NP-40. The cells were then incubated with primary antibodies for 1 h followed by incubation with secondary antibodies for 1 h. The localization of NEMO and LAMP-1 was analysed using a confocal laser-scanning microscope FV100-D (Olympus, Tokyo, Japan). The following antibodies were used: anti-NEMO (sc-8032) and anti-LAMP-1 (sc-5570) (Santa Cruz Biotechnology), Alexa Fluor 488 goat anti-mouse IgG (A11029) and Alexa Fluor 546 goat anti-rabbit IgG (A11035) (Life Technologies). Images in two channels were acquired by sequential scanning. For quantification, a region of interest was defined around an individual cell ( n =30), and the Manders' colocalization coefficients were determined under the same threshold values using FV10-ASW imaging software (Olympus). Statistics Statistically significant differences between the mean values were determined using Student's t -test (*** P <0.01, ** P <0.02 and * P <0.05). Data are presented as the means±s.d. How to cite this article: Shibata, Y. et al . p47 negatively regulates IKK activation by inducing the lysosomal degradation of polyubiquitinated NEMO. Nat. Commun. 3:1061 doi: 10.1038/ncomms2068 (2012).